Controlling the crystalline three-dimensional order in bulk materials by single-wall carbon nanotubes The construction of ordered single-wall carbon nanotube soft-materials at the nanoscale is currently an important challenge in science. Here we use single-wall carbon nanotubes as a tool to gain control over the crystalline ordering of three-dimensional bulk materials composed of suitably functionalized molecular building blocks. We prepare p -type nanofibres from tripeptide and pentapeptide-containing small molecules, which are covalently connected to both carboxylic and electron-donating 9,10-di(1,3-dithiol-2-ylidene)-9,10-dihydroanthracene termini. Adding small amounts of single-wall carbon nanotubes to the so-prepared p -nanofibres together with the externally controlled self assembly by charge screening by means of Ca 2+ results in new and stable single-wall carbon nanotube-based supramolecular gels featuring remarkably long-range internal order. Growing hierarchical architectures at different length scales is at the forefront in science [1] , [2] , [3] , [4] . The well-known correlation between order of materials across different length scales, on one hand, and efficiency of device performance, on the other hand, has fuelled the development of self-organizing small molecules at the nanoscale, the macroscale and so on [5] , [6] , [7] . Despite numerous efforts regarding the construction of well-ordered architectures, the macroscopic control over the three-dimensional (3D) order of bulk materials still remains a key challenge. Such control eases the processability of materials, especially their integration into devices. The incentive is to diminish the number of grain boundaries, on one hand, and macroscopic defects, on the other hand, which act as charge traps and/or affect the device performance [8] , [9] , [10] . A viable strategy to overcome such drawbacks implies the use of liquid crystals. Notably, the fact that liquid crystalline behaviour evolves between isotropic and crystalline phases, facilitates the macroscopic control over the bulk materials and surfaces across all length scales [11] , [12] , [13] . Such advantages are, however, offset by elaborate synthetic protocols and the difficulties to attain liquid crystalline properties. As a matter of fact, developing simpler experimental protocols still remains a major challenge in macroscopic control of the order of bulk materials. In recent years, carbon nanotubes (CNTs), in general, and single-wall CNTs (SWCNT), in particular, have turned into one of the most intriguing nanomaterials because of their unique mechanical and electronic features [14] , [15] . In light of the latter, CNTs are suitable candidates for emerging nanotechnological applications [16] , [17] , [18] , [19] , [20] , [21] . In fact, numerous ways of dispersing CNTs in matrices such as surfactants [22] , polymers [23] , [24] , [25] , biopolymers [26] , [27] , [28] , supramolecular organic gels [29] , [30] and liquid crystals [31] , [32] , [33] , [34] , [35] , [36] were meant to order structures. The use of any of the aforementioned matrices has resulted in hybrid materials, in which both morphology and order are mainly controlled by the matrix components, while CNTs lack any significant role. Thus, the presence of CNTs in, for example, semicrystalline polymeric [37] , [38] and biopolymeric [39] , [40] matrices favours the crystallization of the latter around CNTs. Typically, X-ray diffraction (XRD) experiments performed with the composites reveal d -spacings of the matrix components, which suggests that the incorporation of CNTs into polymer matrices does not provoke sudden changes in the internal structures of the latter. These results correlate with the conformational order of the polymer onto CNT surfaces. On a similar note, in supramolecular gels the presence of CNTs induces gelling processes at concentrations lower than their typical gelling point. However, the lack of XRD data hampers insights into structural changes in the used gel matrix [29] , [30] . 9,10-Di(1,3-dithiol-2-ylidene)-9,10-dihydroanthracenes (exTTFs) have been widely used to form electroactive molecular architectures such as tweezers and tripods, which efficiently interact with CNTs by means of supramolecular interactions. Here important contributions stem from the geometrical complementarity between concave exTTF and convex CNTs [41] . Inspired by the crystallization of semicrystalline polymers in CNT composites, together with the well-documented affinity of the concave geometry of exTTF towards CNTs [42] , [43] , we hypothesized that SWCNTs could be useful additives to control the order of bulk materials. As such, the main goal of the current work is to explore the function of SWCNTs to nucleate long-range order in 3D materials starting from short-range-ordered architectures, particularly exTTF nanostructures ( Fig. 1 ). 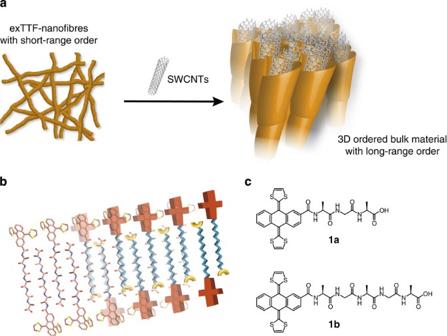Figure 1: 3D bulk materials from peptide-containing exTTFs and SWCNTs. (a) Cartoon showing CNTs as additives for controlling the crystalline ordering in bulk materials. (b) Schematic illustration of a β-sheet secondary supramolecular structure built up by peptide-based exTTFs. (c) Peptide-based exTTFs used in this study. Figure 1: 3D bulk materials from peptide-containing exTTFs and SWCNTs. ( a ) Cartoon showing CNTs as additives for controlling the crystalline ordering in bulk materials. ( b ) Schematic illustration of a β-sheet secondary supramolecular structure built up by peptide-based exTTFs. ( c ) Peptide-based exTTFs used in this study. Full size image For this purpose, two major aspects should be considered; first, CNTs are meant to serve as a template, onto which exTTFs should supramolecularly arrange in an orderly manner ( Fig. 1a,b ). Second, supramolecular arrays of exTTFs and CNTs are expected to be sufficiently stable to transfer their order to the bulk material. Thus, CNTs are used as seeds for growing new ordered 3D bulk materials, which, otherwise, would require more complex protocols. The present approach involves the formation of new 3D exTTF/SWCNTs bulk materials, whose morphologies and order are different from those seen in the individual components. To the best of our knowledge, this aspect is still largely unexplored. Recently, we have reported on a tailored exTTF dipeptide-bearing water-soluble polar dendritic side chains, which efficiently interface with SWCNTs to produce two-dimensional lamellar nanostructures with short-range order [44] . However, the lack of long-range order prompted us to modify the design of peptide-containing exTTFs on two accounts. On one hand, we have extended the peptide chains to ensure both the formation and stabilization of ordered structures involving CNTs and, on the other hand, we have introduced less bulky polar substituents such as carboxylic groups. The latter guarantees not only water solubility but also tuning the resulting 3D morphology and size of the assemblies by charge screening using metal cations. In this work, we demonstrate that SWCNTs are efficient scaffolds to macroscopically control the crystalline ordering in organic bulk materials. To this end, small-angle X-ray scattering (SAXS), XRD and high-resolution transmission electron microscopy (HRTEM) experiments support the notion that the presence of small amounts of SWCNTs are responsible for crystalline ordering of the 3D bulk material at the nanoscale. The sudden changes in the internal structure of the exTTF bulk material take place in the presence of SWCNTs and result, in turn, in remarkable changes in the overall morphology. In particular, new and stable supramolecular gels constituted by long and superhelix fibres with diameters ranging from 40 to 50 nm are formed in the presence of Ca 2+ ions. In these ensembles, SWCNTs are oriented in parallel with respect to the axial axis of the fibre bundle. These experimental findings suggest that SWCNTs are efficiently templating the growth of highly ordered bulk materials. This work represents a valuable example of how SWCNTs effectively control the crystalline ordering in 3D bulk materials stemming from the self-organization of suitably functionalized molecular building blocks ( 1a and 1b ). To the best of our knowledge, the use of SWCNTs as scaffolds to promote the crystalline ordering in bulk materials has barely been explored, despite its great potential for constructing more sophisticated supramolecular ensembles under controlled conditions. Control over the organization of well-ordered p -nanofibres In line with the aforementioned fact, we have designed and synthesized 1a and 1b bearing electron-donating exTTFs, covalently linked to alanyl- and glycyl-rich sequences that carry terminal carboxylic groups. Details on their syntheses and spectroscopic characterization are provided in the Methods section (Synthetic scheme in Supplementary Fig. 1 ). As we have recently reported, exTTF is a versatile building block towards driving the construction and stabilization of well-ordered nanostructures at different length scales [45] , [46] . The presence of short peptides enables the organization of chiral β-sheets as secondary structures [47] , [48] , which ensures the efficient stabilization of a supramolecular order onto SWCNTs. In addition, such organization allows the delocalization of positive charges through stacks of exTTFs. To determine the supramolecular organization of the functionalized molecular building blocks ( 1a and 1b ), we have carried out a variety of complementary spectroscopic and microscopic investigations. 1a gave rise under soft basic conditions (NaHCO 3 solutions at pH 9) to the diagnostic absorption band of π–π interacting exTTFs at around 490 nm [42] , [43] ( Fig. 2a ). The originally seen absorption bands of pristine exTTFs were, however, recovered after either applying heat or the addition of methanol, which attests the reversibility of the process ( Supplementary Fig. 2A–C ). In the case of 1b , the 490 nm diagnostic band is observed at both soft basic conditions and at physiological pH ( Fig. 2b ). Similar to 1a , this process was found to be reversible when either applying heat or the addition of methanol ( Supplementary Fig. 2D,E ). 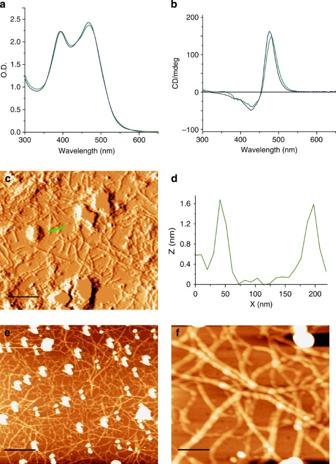Figure 2: Ultraviolet–visible, CD spectra and AFM for thep-nanofibres. (a) Absorption spectra of1a(green line) and1b(blue line) at 2 × 10−3M both in aqueous solution under soft basic conditions (pH 8–9). (b) CD spectra of1a(green line) and1b(blue line) at 2 × 10−3M both in aqueous solution under soft basic conditions (pH 8–9). (c) AFM image of1adeposited under soft basic conditions (pH 8–9) onto mica. Scale bar, 500 nm. (d) Height profile across the green line inc. (e) AFM image of1bdeposited at physiological pH onto mica. Scale bar, 1,000 nm. (f) Magnification of image (e). Scale bar, 220 nm. Figure 2: Ultraviolet–visible, CD spectra and AFM for the p -nanofibres. ( a ) Absorption spectra of 1a (green line) and 1b (blue line) at 2 × 10 −3 M both in aqueous solution under soft basic conditions (pH 8–9). ( b ) CD spectra of 1a (green line) and 1b (blue line) at 2 × 10 −3 M both in aqueous solution under soft basic conditions (pH 8–9). ( c ) AFM image of 1a deposited under soft basic conditions (pH 8–9) onto mica. Scale bar, 500 nm. ( d ) Height profile across the green line in c . ( e ) AFM image of 1b deposited at physiological pH onto mica. Scale bar, 1,000 nm. ( f ) Magnification of image ( e ). Scale bar, 220 nm. Full size image Circular dichroism (CD) assays carried out with 1a , under soft basic conditions, led to a strong bisignate signal with a positive Cotton effect at 480 nm, a negative Cotton effect at 431 nm and a zero cross point at 456 nm ( Fig. 2b and Supplementary Fig. 2F ). The strong ellipticity observed under these experimental conditions suggests a major ordering of π–π-interacting exTTFs in the form of chiral arrays. In addition, XRD experiments support for 1a the existence of well-defined β sheets ( Supplementary Fig. 3A ). Similar to that observed for 1a , CD experiments with 1b indicate the presence of strong bisignated signals all the way up to 90 °C ( Fig. 2b and Supplementary Fig. 2G,H ). In accordance with the results stemming from absorption spectroscopy, these signals were present under both physiological and soft basic conditions. Similar to 1a , XRD experiments confirm the exclusive presence of β-sheet type structures ( Supplementary Fig. 3B ). Atomic force microscopy (AFM) inspections carried out with 1a and 1b supported the existence of curved rope-like nanofibres with average diameters of 1.5 nm and twisted shapes ( Fig. 2c–f ). In summary, exTTF derivatives of tripeptide 1a and pentapeptide 1b self-organize at the nanoscale to yield twisted p -type nanofibres similar to those recently reported [45] , [46] . In addition, in both cases, XRD and CD experiments ( Supplementary Fig. 3C–E ) support that the corresponding p -type nanofibres are composed of stacked β sheets with a short-range order at d -spacings of 2 θ =10° and 20°, which is typical for β-sheet arrangements. Formation of n / p -nanocomposite hydrogels In the search for 3D bulk long-range-ordered materials by simple experimental procedures, we used SWCNTs as additives to macroscopically control the order of the exTTF nanofibres in the 3D bulk material. The addition of small amounts of SWCNTs was expected to induce long-range order in the 3D bulk material, at larger distances than those observed for each of its individual components. Here we realized stable gels by the addition of a saturated CaCl 2 solution to a concentrated soft basic solution of 1a or 1b (>5 × 10 −3 M with 7.5 equivalents of NaHCO 3 ) in the presence of SWCNTs. The latter were dispersed by sonication with concentrations lower than 0.2 wt% (refs 26 , 49 , 50 ; for full details, see Methods section). A thorough characterization of the attained bulk material has been performed by scanning electron microscopy (SEM), TEM, HRTEM, XRD and SAXS measurements. Interestingly, SEM images revealed the presence of large fibres with diameters ranging from 40 to 50 nm for 1a and 1b in the presence of SWCNTs and CaCl 2 ( Supplementary Fig. 4C–F ). In addition, in the case of 1b/ SWCNTs/CaCl 2 the presence of left-handed superhelixes with similar diameters was also clearly observed ( Fig. 3a ). 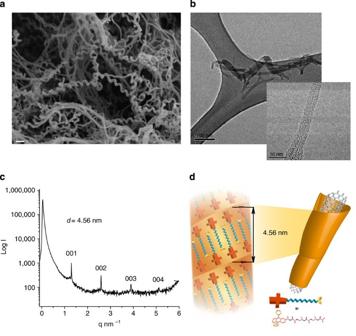Figure 3: Electron microscopy, SAXS and schematic illustration ofn/p-nanocomposite hydrogels. (a) SEM image of the xerogel obtained for1b/SWCNT on treating with CaCl2. Scale bar, 200 nm. (b) TEM image of the xerogel obtained for1b/SWCNT. Scale bar, 100 nm. Inset: HRTEM image of the xerogel obtained for1b/SWCNT gel. Scale bar, 10 nm. (c) SAXS pattern of the xerogel obtained for1b/SWCNT. (d) Schematic illustration depicting the lamellar packing of exTTF1baround SWCNTs. Figure 3: Electron microscopy, SAXS and schematic illustration of n / p -nanocomposite hydrogels. ( a ) SEM image of the xerogel obtained for 1b /SWCNT on treating with CaCl 2 . Scale bar, 200 nm. ( b ) TEM image of the xerogel obtained for 1b /SWCNT. Scale bar, 100 nm. Inset: HRTEM image of the xerogel obtained for 1b /SWCNT gel. Scale bar, 10 nm. ( c ) SAXS pattern of the xerogel obtained for 1b /SWCNT. ( d ) Schematic illustration depicting the lamellar packing of exTTF 1b around SWCNTs. Full size image In control experiments, gels formed from 1a and 1b in the absence of SWCNTs led to a substantially different picture ( Supplementary Fig. 4A,B ). In fact, SEM images taken for gels of 1a and 1b in the presence of CaCl 2 failed to imply neither left-handed superhelixes nor any straight fibres. Instead, only soft curved fibres were discernable. In both cases, SAXS experiments are in agreement with the lack of long-range order in the bulk material ( Supplementary Fig. 5A,C ), and only the typical β-sheet reflections at distances around 9.8 and 4.5 Å were observed in XRD experiments. In complementary TEM investigations ( Supplementary Fig. 6 ), the presence of SWCNTs and CaCl 2 revealed the existence of domains with large straight and superhelix fibres in the case of 1b /SWCNT/CaCl 2 ( Supplementary Fig. 6A,B )—a finding that is in agreement with the SEM investigations. In addition, homogenous small straight bundles with diameters ranging from 3 to 10 nm are observed in the area of such domains ( Supplementary Fig. 7A–E ). HRTEM images of such bundles prompt to the fact that they are formed by few SWCNTs, which are surrounded by organic materials ( Supplementary Fig. 7F–I ). It is worth mentioning that SWCNTs are placed here parallel to the axial axis of the fibre bundles, which corroborates the templating role of SWCNTs in the overall construction of such fibres. Furthermore, the distances observed between individual CNTs ranged from 0.6 to 1.1 nm. These observations support the notion that SWCNTs, placed within the organic matrix, induce morphology in the bulk material that is substantially different from that of its individual components. In addition, it is worth mentioning the absence of randomly SWCNT bundles sticking out of the organic matrix. We consider this fact as strong evidence for an efficient interfacing between exTTFs and SWCNTs. Energy-dispersive X-ray analyses confirmed the presence of carbon, sulphur, calcium and chloride ( Supplementary Fig. 6E ). To determine whether the changes of the bulk material morphology observed in the presence of SWCNTs involved a sudden change of its internal structure, we carried out complementary SAXS and XRD experiments. SAXS experiments with the 1a /SWCNT/CaCl 2 gel, which did not give rise to any appreciable peaks in the zone of the matrix component, infer the lack of order in the bulk material. Furthermore, no peaks for the typical d -spacings of β sheets were observed in the XRD experiments ( Supplementary Fig. 5D,E ). These experimental findings correlate with the shorter peptide chain, which results in a lower stability of the exTTF supramolecular structures as they are formed at the surface of SWCNTs, and, which prevents the induced order in the bulk material. As it will be shown later, this behaviour is in agreement with the inversion and loss of ellipticity observed for 1a in the presence of SWCNTs by means of CD. In sharp contrast, in SAXS experiments with the 1b /SWCNT/CaCl 2 gel, up to four peaks corresponding to lamellar packing with a periodical d -spacing of 4.56 nm are discernable ( Fig. 3c ). The latter indicates the presence of long-range order in the bulk material. Please note that such a long-range order is new and inherent for the formed bulk material and it was not observed in any of the individual components. As mentioned before, HRTEM inspection of the bulk material from 1b in the presence of SWCNTs showed that the distances between SWCNTs ranged from 0.5 to 1.1 nm. Therefore, the origin of the lamellar packing observed in SAXS experiments with 1b /SWCNT/CaCl 2 must stem from other types of supramolecular order. As a matter of fact, we postulate that the lamellar packing relates to the organization of exTTF 1b around SWCNTs ( Fig. 3d ). Please note that the presence of well-defined and sharpened peaks, with four reflection planes in the SAXS experiments, corroborates the presence of a highly ordered nanocomposite. At this point, it is safe to conclude that the presence of SWCNTs in form of additives induces a new ordered exTTF 3D bulk material, which is completely different in terms of internal structure and morphology from that observed in the absence of SWCNTs. In addition, the presence of SWCNTs in the material causes a crystalline ordering of the exTTF matrix at the nanoscale, which is otherwise not observed. Furthermore, the typical β-sheet reflections in XRD experiments with the bulk material in the presence of SWCNTs demonstrated that the internal exTTF order is not disrupted by the presence of CNTs ( Supplementary Fig. 5B ). Interfacing between p -nanostructures and SWCNTs Considering the aforementioned ability of SWCNTs as additives to macroscopically control the 3D-ordered exTTF bulk materials, we carried out a detailed study on the interfacing between exTTF p -nanostructures—used as matrix components—and SWCNTs. This study should allow establishing the relationship between the stability of the exTTF p -nanostructures and the crystalline order of the bulk material in the presence of SWCNTs, as well as documenting the impact of the latter on the stabilization of the photogenerated charge-separated state. We tested the nanofibres formed from 1a and 1b as wrapping agents for SWCNTs. First insights into mutually interacting components came from absorption spectroscopy with focus on the exTTF absorption characteristics. Interestingly, 1a and 1b dispersed SWCNTs reasonably well in aqueous solutions. When using nanofibres— 1a and 1b both under soft basic conditions (pH 8–9)—to wrap around SWCNTs, the 490-nm absorption decreased in intensity and red shifted by nearly 10 nm in the presence of SWCNTs ( Fig. 4a,b ). Implicit in this bathochromic shift is the successful wrapping of the nanofibres around SWCNTs. 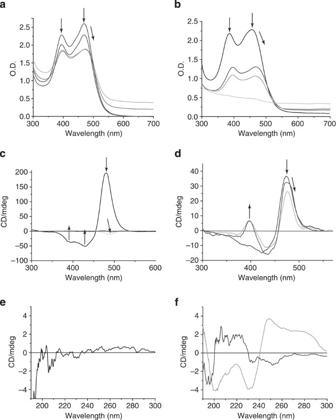Figure 4: Ultraviolet and CD experiments forp-nanostructures/SWCNTs. (a) Absorption assay of1a(1.3 × 10−4M) under soft basic conditions (pH 8–9) with SWCNTs (suspension of 1–2 mg in 0.5 ml of tetrahydrofuran (THF))—please see arrows for progression. (b) Absorption assays of1b(1.3 × 10−4M) under soft basic conditions (pH 8–9) with SWCNTs (suspension of 1–2 mg in 0.5 ml of THF)—please see arrows for progression. (c) CD assay ofp-nanofibres (1a) under soft basic conditions (pH 8–9) with SWCNTs—please see arrows for progression. (d) CD assay ofp-nanofibres (1b) under soft basic conditions (pH 8–9) with SWCNTs—please see arrows for progression. (e) Peptide zone of CD of1aunder soft basic conditions (pH 8–9) with SWCNTs. (f) Peptide zone of CD of1bunder soft basic conditions (pH 8–9) immediately on addition of SWCNTs (black line) and 15 min later (grey line). Please note that no significant changes in the ultraviolet–visible spectrum occur in the 190–300-nm range and, as such, are omitted. Figure 4: Ultraviolet and CD experiments for p -nanostructures/SWCNTs. ( a ) Absorption assay of 1a (1.3 × 10 −4 M) under soft basic conditions (pH 8–9) with SWCNTs (suspension of 1–2 mg in 0.5 ml of tetrahydrofuran (THF))—please see arrows for progression. ( b ) Absorption assays of 1b (1.3 × 10 −4 M) under soft basic conditions (pH 8–9) with SWCNTs (suspension of 1–2 mg in 0.5 ml of THF)—please see arrows for progression. ( c ) CD assay of p -nanofibres ( 1a ) under soft basic conditions (pH 8–9) with SWCNTs—please see arrows for progression. ( d ) CD assay of p -nanofibres ( 1b ) under soft basic conditions (pH 8–9) with SWCNTs—please see arrows for progression. ( e ) Peptide zone of CD of 1a under soft basic conditions (pH 8–9) with SWCNTs. ( f ) Peptide zone of CD of 1b under soft basic conditions (pH 8–9) immediately on addition of SWCNTs (black line) and 15 min later (grey line). Please note that no significant changes in the ultraviolet–visible spectrum occur in the 190–300-nm range and, as such, are omitted. Full size image Complementary CD titrations ( Fig. 4c ) showed that when titrating 1a with SWCNTs the bisignate signals of the exTTF nanostructures progressively decrease with the concomitant formation of a new, red-shifted bisignate signal. Importantly, the latter signal reveals an opposite helical handedness relative to the initial signal. It is worth mentioning that similar inversions have previously been observed for supramolecular [51] and covalent helical polymers [52] under certain external stimuli. Please note that, in the presence of SWCNTs, the typical β-sheet signatures in the CD spectra disappeared ( Fig. 4e ). These experimental findings suggest some kinetic instability stemming from the presence of SWCNTs in the case of 1a . This is also confirmed by the strong decreasing ellipticity and the inversion of the handedness observed for the bisignate signal. On the other hand, CD titrations carried out with 1b and SWCNTs gave rise to a partial depletion of the bisignate signals of the exTTF nanostructures and the formation of a red-shifted bisignate signal, but in this case without helical inversion. These experimental observations support the notion of an efficient wrapping of the exTTF nanostructures around SWCNTs, without losing their helical ordering ( Fig. 4d ). Moreover, the typical β-sheet signatures are still present in 1b /SWCNT and transform into a more complex CD spectrum after a short period of 15 min ( Fig. 4f ). Similar are the results that emerged when focusing on the absorption of SWCNTs. Here the features of the E 11 absorption peaks of SWCNTs red shift from 980, 1,025, 1,155 and 1,265 nm in the case of sodium dodecyl benzene sulphonate (SDBS)/SWCNT to 1,006, 1,052, 1,156 and 1,292 nm in the case of 1a /SWCNT ( Supplementary Fig. 8A ). On the other hand, the E 22 absorption peaks in SDBS/SWCNT at 450, 500, 570, 590, 650 and 725 nm were only marginally affected by the presence of 1a with red shifts that are on the order of a few nanometres. For 1b /SWCNT, maxima evolved at 1,006, 1,054, 1,150 and 1,290 nm ( Supplementary Fig. 8B ). Insights into exTTF/SWCNT ground-state electronic interactions came from Raman experiments. Here the three most important signatures, that is, RBM-, D- and G modes, reveal upshifts in D 2 O suspensions of SDBS/SWCNT with respect to 1a /SWCNT as well as in the solid without evidencing losses in resonance. For example, the G mode shifts from 1,590±2 to 1,592±2 and 1,591±2 cm −1 in the presence of 1a and 1b , respectively ( Supplementary Fig. 8C,D ). This indicates the fact that π–π interactions are operative between 1a or 1b and SWCNTs. Augmentation through ground-state charge transfer/doping seem to play, however, only a minor role. Turning to AFM assays, the images are best described as homogenous distributions of nanofibre/SWCNT nanohybrids— 1a /SWCNT and 1b /SWCNT. A closer inspection reveals, nevertheless, that SWCNTs are uniformly covered with nanofibres of 1a and 1b ( Fig. 5a–d and Supplementary Fig. 9 ). Analyses of individual nanohybrids by means of AFM confirmed heights of around 2.3–2.8 nm for 1a and 3.5–4 nm for 1b . 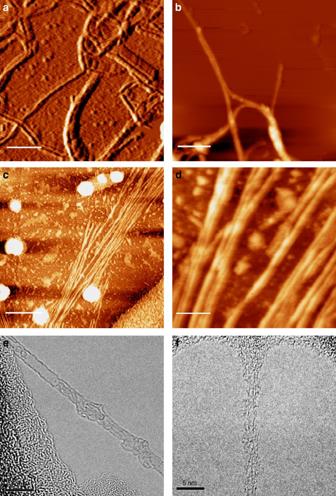Figure 5: Microscopy characterization for1a/SWCNTs and1b/SWCNTs. (a) AFM phase image of1a/SWCNTs deposited under soft basic conditions (pH 8–9) onto mica. Scale bar, 130 nm. (b) AFM image of1a/SWCNT deposited under soft basic conditions (pH 8–9) onto highly ordered pyrolytic graphite (HOPG). Scale bar, 120 nm. (c) AFM image of1b/SWCNT deposited under soft basic conditions (pH 8–9) onto HOPG. Scale bar, 960 nm. (d) Amplification of 5C showing the homogenous wrapping ofp-nanofibres around SWCNTs. Scale bar, 180 nm. (e) HRTEM image of1a/SWCNT drop-casted under soft basic conditions (pH 8–9) onto TEM grids. Scale bar, 5 nm. (f) HRTEM image of1b/SWCNT drop-casted under soft basic conditions (pH 8–9) onto TEM grids. Scale bar, 5 nm. Figure 5: Microscopy characterization for 1a /SWCNTs and 1b /SWCNTs. ( a ) AFM phase image of 1a /SWCNTs deposited under soft basic conditions (pH 8–9) onto mica. Scale bar, 130 nm. ( b ) AFM image of 1a /SWCNT deposited under soft basic conditions (pH 8–9) onto highly ordered pyrolytic graphite (HOPG). Scale bar, 120 nm. ( c ) AFM image of 1b /SWCNT deposited under soft basic conditions (pH 8–9) onto HOPG. Scale bar, 960 nm. ( d ) Amplification of 5C showing the homogenous wrapping of p -nanofibres around SWCNTs. Scale bar, 180 nm. ( e ) HRTEM image of 1a /SWCNT drop-casted under soft basic conditions (pH 8–9) onto TEM grids. Scale bar, 5 nm. ( f ) HRTEM image of 1b /SWCNT drop-casted under soft basic conditions (pH 8–9) onto TEM grids. Scale bar, 5 nm. Full size image Taking the average diameter of the rope-like nanofibres of 1.5 nm into account, diameters of 2.5–2.8 nm are in accordance with the presence of individual SWCNTs, which are wrapped by nanofibres. By the same token, the height histogram, which features maxima at 2.5 nm and onsets at around 6.0 nm, confirms the coexistence of mostly individualized 1a /SWCNT and/or 1b /SWCNT with small clusters ( Supplementary Fig. 9 ). With the use of TEM, the coexistence of individualized SWCNTs and of loosened bundles was further attested ( Supplementary Fig. 10 ). Clearly, the nanohybrids possess a different organization when compared with random bundles of pristine SWCNTs. In agreement with the AFM images, HRTEM images attest the homogenous coverage of SWCNTs ( Fig. 5e,f ). As a driving force for the latter, we assume that p / n interactions are at work between exTTF nanofibres and SWCNTs. The fluorescence of 1a /SWCNT under soft basic conditions (pH 8–9) evolves at 1,003, 1,069, 1,172 and 1,311 nm ( Supplementary Fig. 11A,B ). They are in the same way red shifted as seen for the absorption features— vide supra . For example, the corresponding maxima appear for SDBS/SWCNT at 958, 1,028, 1,125 and 1,250 nm, which are attributed to (6,5), (7,5), (7,6) and (8,7) SWCNTs. When comparing the fluorescence intensity of 1a /SWCNT with that of SDBS/SWCNT exhibiting both equal absorbances at the excitation wavelength, a significant quenching is noted. In 1a /SWCNT, the quenching is as strong as 99% ( Supplementary Fig. 11E ). When inspecting the fluorescence of 1b /SWCNT rather than that of 1a /SWCNT, the overall quenching is 95% ( Supplementary Fig. 11C,D,F ). The fluorescence assays were complemented by transient absorption spectroscopy to determine the dynamics of the ultrafast singlet excited-state deactivation in 1a /SWCNT as well as 1b /SWCNT and to characterize the products evolving from interacting of 1a and 1b p -nanofibres with SWCNTs. We started our investigations with SDBS/SWCNT reference experiments. The baseline is, in the case of SDBS/SWCNT, replaced with a strong bleaching that dominates the differential absorption spectra throughout the visible and near-infrared (NIR) regions. The major minima are seen at 570, 590, 650, 725, 985 and 1,130 nm in addition to shoulders at 1,025 and 1,270 nm and a maximum at 1,465 nm. Multiwavelength analyses of the bleaching characteristics resulted in complex dynamics with two dominant lifetimes, namely, 0.6 and 68 ps (ref. 43 ). In control experiments, 1a and 1b were probed by photoexcitation at 387 nm ( Supplementary Fig. 12A,B ). In particular, exTTF-centred excited states evolve featuring spectral characteristics that include transient maxima around 470, 600 and 920 nm for 1a , and 574, 615 and 820 nm as well as a transient bleaching at 465 nm for 1b . The lifetimes are, however, less than 2±1 ps in both cases—a fact that correlates with a strong second-order vibronic spin orbit coupling. Following photoexcitation of 1a /SWCNT at 387 nm, we see in line with the absorption spectra the rapid formation of transient maxima at 465, 545 and 680 nm as well as transient bleaching at 1,040 and 1,145 nm that substantiates the excitation of 1a and SWCNTs, respectively ( Supplementary Fig. 12C–E ). Notable are also red shifts of the differential absorption changes when compared with SDBS/SWCNT [43] . Such a trend mirror images the differences in the absorption spectra of 1a /SWCNT and SDBS/SWCNT. In general, the photoexcited exTTF and SWCNT states are in 1a /SWCNT shorter lived and transform with a lifetime of 1.4±0.3 ps into a new transient. In the visible, the newly formed transient is characterized by a broad maximum at 680 nm. The latter resembles the radiolytically and photolytically generated fingerprint of the one electron-oxidized radical cation of exTTF [53] , [54] . In the NIR, appreciable blue shifts of the transient bleaching are detected, with minima that shift from 1,040 and 1,145 nm to 1,010 and 1,135 nm, respectively, followed by a broad transient between 1,150 and 1,600 nm. Implicit are new conduction band electrons—injected from the exTTF—shifting the transitions to lower energies. As a matter of fact, we reach the conclusion that the selective excitation of 1a /SWCNT, in which sizeable shifts of electron density prevail even in the ground state, is followed by a full separation of charges. The latter infers oxidation of exTTF and reduction of SWCNTs. By following the characteristics of the oxidized exTTF and the reduced SWCNTs, we deduce a lifetime of the electron transfer product of 125±20 ps. Fairly similar are the differential absorption changes in the NIR on photoexcitation of 1b /SWCNT at 387 nm. A marked difference is seen, however, in the visible. In particular, transient bleaching in the range of absorptive transitions of semiconducting SWCNTs at 590 and 650 nm dominate the exTTF features. Nevertheless, also in 1b /SWCNT the photoexcited exTTF and SWCNT states are short lived with lifetimes of 15±0.3 ps ( Supplementary Fig. 12F–H ). The product of the excited-state decay is attributed to oxidized exTTF and reduced SWCNTs. When turning to the lifetime of the electron transfer product in 1b /SWCNT, it is longer lived than in 1a /SWCNT with a lifetime of 210±10 ps. The presence of carboxylates and Na + —from the basic soft conditions—complexes might influence the highest occupied molecular orbital/lowest unoccupied molecular orbita levels of the corresponding electroactive species, namely, exTTF and SWCNTs, or might even interact with them through anion–π or cation–π interactions [55] , [56] . However, our investigations reveal that on photoexcitation, localized exTTF- and SWCNT-excited states evolve and transform rapidly into well-characterized electron transfer products ruling out any major impact. General methods 1 H NMR and 13 C NMR spectra were recorded on a Bruker Avance-300 or a Bruker Avance AMX-700. Unless otherwise indicated, chemical shifts are reported in p.p.m. downfield from tetramethylsilane at room temperature using deuterated solvents as an internal standard. Abbreviations used for splitting patterns are s=singlet, br s=broad singlet, d=doublet, t=triplet q=quadruplet and m=multiplet. Matrix-assisted laser desorption ionization (MALDI) high-resolution mass spectrometry (MS) was performed on a MAT 95 thermo spectrometer using trans -2-[3-(4-tert-Butylphenyl)-2-methyl-2-propenylidene]malononitrile matrix. Column chromatography was carried out on Merck silica gel 60 (70–230 mesh). All solvents were dried by means of standard protocols with sodium and benzophenone as indicator. HiPCO and CoMoCAT SWCNTs were purchase from Carbon Nanotechnologies and Southwest Nanotechnologies, respectively, and used without any further purification treatment. Other reagents were purchased from Sigma-Aldrich and were used without further purification. CD measurements were carried out on a JASCO J-815 DC spectrometer. Absorption spectra were recorded with a Varian Cary 50 and 5000 spectrophotometer and UV-3600 Shimadzu ultraviolet–visible–NIR spectrophotometer. Steady-state fluorescence spectra were acquired by a FluoroLog3 spectrometer (Horiba) with a IGA Symphony (512 × 1 × 1 μm 3 ) detector in the NIR detection range. Transient absorption spectroscopy was performed with 387 nm laser pulses from an amplified Ti/sapphire laser system (ModelCPA2101, Clark-MXR Inc.; output: 775 nm, 1 kHz and 150 fs pulse width) in the Transient Absorption Pump/Probe System Helios from Ultrafast Systems with 200 nJ laser energy. Raman spectra were with a Fourier transform–Raman spectrometer RFS100 from Bruker with an excitation wavelength of 1,064 nm and a liquid nitrogen-cooled germanium detector. Synthesis and characterization A synthetic scheme is provided in Supplementary Fig.1 . N-(tert-Butoxycarbonyl)- L -alanyl-glycyl- L -alanine ethyl ester ( 2 ): To a solution of N -( tert -butoxycarbonyl)- L -alanyl-glycine [57] (500 mg, 2.03 mmol) in dry N,N -dimethylformamide (DMF) (20 ml), O -benzotriazole- N , N , N ′, N ′-tetramethyl-uronium-hexafluoro-phosphate (1.16 g, 3.05 mmol) and N,N -diisopropylethylamine (1.1 ml, 6.09 mmol) were added under argon flow at room temperature. After 5 min of activation, L -alanine ethyl ester hydrochloride (406 mg, 2.64 mmol) was added and the reaction mixture was stirred for 3 h. The solvent was removed under reduced pressure and the residue was redissolved in CH 2 Cl 2 (30 ml) and washed with a saturated Na 2 CO 3 aqueous solution (3 × 10 ml) and a saturated NH 4 Cl aqueous solution (3 × 10 ml) and the organic layer was dried over Na 2 SO 4 . The solvent was removed under reduced pressure to obtain 2 as a brown oil with enough purity to be used in the next reaction (745 mg, 96%); 1 H NMR (300 MHz, CDCl 3 ): δ 7.37 (br s, 1H), 7.24 (br s, 1H), 5.41 (br s, 1H), 4.48 (m, 1H), 4.19–4.08 (m, 3H), 4.08–3.79 (m, 2H), 1.38 (d, 3 J =7 Hz, 2H), 1.38 (s, 9H), 1.33 (d, 3 J =7 Hz, 2H), 1.22 (t, 3 J =7 Hz, 3H); 13 C NMR (75 MHz, CDCl 3 ): δ 172.9, 172.1, 170.1, 158.1, 80.7, 61.8, 49.6, 48.4, 43.1, 28.4, 18.3, 17.4, 14.7; HRMS electrospray ionization (ESI; m / z ): [M+H] + calcd. for C 15 H 28 N 3 O 6 , 346.1972; found, 346.1986. L -Alanyl-glycyl- L -alanine ethyl ester hydrochloride ( 3 ): To a solution of 2 (550 mg, 1.44 mmol) in dry CH 2 Cl 2 (4 ml), a solution of HCl 2 M in diethyl ether (1 ml) was added and the reaction mixture was stirred under argon flow for 24 h. Reaction was monitored by TLC using ninhydrin as a revealing agent. The solvent was evaporated at reduced pressure and the residue was redissolved in the minimum volume of methanol for being precipitated by adding cold diethyl ether. Product 3 was obtained as a colourless oil after centrifugation (350 mg, 86%). 1 H NMR (300 MHz, CD 3 OD): δ 4.40 (q, 3 J =7 Hz, 1H), 4.17 (q, 2H), 4.03–3.92 (m, 3H), 1.53 (d, 3 J =7 Hz, 3H), 1.39 (d, 3 J =7.3 Hz, 3H), 1.26 (t, 3 J =7 Hz, 3H); 13 C NMR (75 MHz, CD 3 OD): δ 174.2, 171.6, 170.8, 62.5, 50.4, 49.5, 43.2, 17.8, 17.6, 14.5; HRMS (ESI; m / z ): [M+H] + calcd. for C 10 H 20 N 3 O 4 , 246.1448; found, 246.1454. L -Alanyl-glycyl- L -alanyl-glycyl- L -alanine hydrochloride ( 4 ): Standard solid phase hydroxymethyl-based resin procedure was used to synthesize the desired pentapeptide sequence 4 with a free amine and carboxylic acid groups at the N-terminus and C-terminus positions, respectively [58] . A Wang resin preloaded with Fmoc- L -alanine was used, minimizing epimerization and dipeptide formation; [ α ] D =−24.8 (0.029 M in methanol); 1 H NMR (300 MHz, CD 3 OD): δ 4.49–4.30 (m, 2H), 4.04–3.86 (m, 5H), 3.72 (s, 3H), 1.54 (d, 3 J =7.1 Hz, 3H), 1.40 (d, 3 J =7.3 Hz, 6H); 13 C NMR (75 MHz, CD 3 OD): δ 175.9, 175.4, 171.7, 171.2, 171.1, 50.9, 50.3, 49.4, 43.4, 43.3, 17.7, 17.4; HRMS (ESI; m / z ): [M+H] + calcd. for C 13 H 24 N 5 O 6 , 346.1721; found, 346.1727. L -Alanyl-glycyl- L -alanyl-glycyl- L -alanine methyl ester hydrochloride ( 5 ): To a solution of 4 (140 mg, 0.37 mmol) in methanol (5 ml), 1.8 ml of a solution of trimethylsilyldiazomethane (3.6 mmol) in hexane (2.0 M) was added dropwise. The mixture was allowed to react over 30 min at room temperature. The solvent was evaporated at reduced pressure and the residue was redissolved in the minimum volume of methanol. Precipitation of the product was carried out by adding cold diethyl ether. After centrifugation, product 5 was obtained as a white solid (127 mg, 87%); [ α ] D =−34.5 (0.028 M in methanol); 1 H NMR (300 MHz, CD 3 OD): δ 4.46–4.27 (m, 2H), 4.06–3.82 (m, 5H), 1.53 (d, 3 J =7.1 Hz, 3H), 1.40 (d, 3 J =7.2 Hz, 3H), 1.39 (d, 3 J =6.9 Hz, 3H); 13 C NMR (75 MHz, CD 3 OD): δ 173.7, 173.4, 171.7, 171.2, 171.1, 50.9, 50.3, 49.4, 48.1, 43.4, 43.3, 17.7, 17.1; HRMS (ESI; m / z ): [M+H] + calcd. for C 14 H 26 N 5 O 6 , 360.1877; found, 360.1888. N-[9,10-Di(1,3-dithiol-2-ylidene)-9,10-dihydroanthracene-2-carbonyl]- L -alanyl-glycyl- L -alanine ethyl ester ( 6 ): To a solution of 9,10-di(1,3-dithiol-2-ylidene)-9,10-dihydroanthracene-2-carboxylic acid (exTTF-COOH) [46] (30 mg, 71 μmol), 3 (26 mg, 92 μmol) and N,N -diisopropylethylamine (40 μl, 213 μmol) in dry DMF (7 ml), O -benzotriazole- N , N , N ′, N ′-tetramethyl-uronium-hexafluoro-phosphate (42 mg, 107 μmol) was added at room temperature under argon flow. The resultant mixture was stirred under argon for 1 h. The solvent was evaporated at reduced pressure and the residue was subjected to column chromatography (eluent: CH 2 Cl 2 /CH 3 OH 25:1, v/v). Product 6 was precipitated in hexane and it was obtained as a bright orange powder (35 mg, 76%). 1 H NMR (700 MHz, CDCl 3 ): δ 8.18 (s, 1H), 7.79–7.68 (m, 4H), 7.38–7.31 (m, 2H), 7.14–7.05 (br s, 1H), 7.05–6.94 (m, 1H), 6.87 (d, 3 J =6.5 Hz, 1H), 6.37–6.32 (m, 4H), 4.75–4.63 (m, 1H,), 4.62–4.51 (m, 1H), 4.25–4.12 (m, 3H), 3.92 (m, 1H), 1.58 (d, 3 J =7 Hz, 3H), 1.50–1.43 (m, 3H), 1.25 (t, 3 J =7 Hz, 3H); 13 C NMR (175 MHz, CDCl 3 ): δ 172.9, 172.8, 168.3, 167.2, 138.7, 138.2, 135.8, 135.1, 135.0, 126.2, 125.1, 124.9, 124.6, 123.8, 117.4, 117.3, 117.1, 61.6, 49.9, 48.3, 43.1, 18.1, 17.9, 14.1; HRMS (MALDI; m / z ): [M] + calcd. for C 31 H 29 N 3 O 5 S 4 , 651.0985; found, 651.0984. N-[9,10-Di(1,3-dithiol-2-ylidene)-9,10-dihydroanthracene-2-carbonyl]- L -alanyl-glycyl- L -alanyl-glycyl- L -alanine methyl ester ( 7 ): To a solution of exTTF-COOH (45 mg, 0.106 mmol) in dry CH 2 Cl 2 (15 ml), ethyl(dimethylaminopropyl)carbodiimide (61 mg, 0.318 mmol) and 4-dimethylaminopyridine (2 mg, 16 μmol) were added at −15 °C under argon flow. After 5 min of activation, 5 (50 mg, 0.106 mmol) was added dissolved in dry DMF (3 ml). The reaction mixture was allowed to stir at room temperature for 2 h. The mixture was washed with a saturated NH 4 Cl aqueous solution (3 × 10 ml) and the organic layer was dried over Na 2 SO 4 . The residue was subjected to neutral aluminium oxide column chromatography (eluent: CH 2 Cl 2 /ethanol, 20:1, v-v). The solvent was removed under reduced pressure to yield 7 as a bright orange powder (62 mg, 76%). 1 H NMR (500 MHz, CD 3 OD): δ 8.25 (s, 1H), 7.83 (dd, 3 J =8 Hz, 3 J =1.6 Hz, 1H), 7.79–7.74 (m, 1H), 7.72–7.67 (m, 2H), 7.32–7.27 (m, 2H), 6.53–6.44 (m, 4H), 4.55–4.47 (m, 1H), 4.46–4.30 (m, 2H), 4.05–3.94 (m, 2H), 3.89–3.80 (m, 2H), 3.69 (s, 3H), 1.54 (d, 3 J =7 Hz, 3H), 1.52–1.46 (m, 3H), 1.35 (d, 3 J =7 Hz, 3H); 13 C NMR (125 MHz, CD 3 OD): δ 174.5, 173.5, 170.9, 170.3, 139.1, 136.1, 135.6, 135.5, 130.7, 126.2 (2), 125.1, 125.0, 124.6, 120.9, 117.7, 117.5, 51.8, 51.2, 50.0, 48.6, 42.9, 42.4, 16.5 (2), 16.4; HRMS (MALDI; m / z ): [M] + calcd. for C 35 H 35 N 5 O 7 S 4 , 765.1414; found, 765.1397. N-[9,10-Di(1,3-dithiol-2-ylidene)-9,10-dihydroanthracene-2-carbonyl]- L -alanyl-glycyl- L -alanine ( 1a ): The compound 6 (50 mg, 0.09 mmol) was added to a solution of KOH 0.2 M in ethanol/H 2 O (9:1, v-v; 8 ml). The mixture reaction was stirred for 120 min at room temperature. After addition of hydrochloric acid until aqueous solution became neutral, the product was extracted with CH 2 Cl 2 (3 × 20 ml). The combined organic layers were dried over Na 2 SO 4 before the solvent was removed in vacuum to yield final product 1a as an orange powder (48 mg, 98%). 1 H NMR (500 MHz, CD 3 OD): δ 8.25 (s, 1H), 7.85–7.75 (m, 2H), 7.74–7.68 (m, 2H), 7.32–7.28 (m, 2H), 6.50 (s, 1H), 6.48 (s, 1H), 4.54 (q, 3 J =7 Hz, 1H), 4.48–4.39 (m, 1H), 4.05–3.83 (m, 2H), 1.57–1.50 (m, 6H); 13 C NMR (125 MHz, CD 3 OD): δ 175.0 (2), 170.2, 168.6, 139.0, 138.9, 136.1, 135.7, 135.6, 131.1, 126.2, 126.1, 125.1, 125.0, 124.9, 124.6, 121.0, 117.4, 117.3, 49.9, 48.3, 42.5, 16.6; HRMS (MALDI; m / z ): [M] + calcd. for C 29 H 25 N 3 O 5 S 4 , 623.0672; found, 623.0686. N-[9,10-Di(1,3-dithiol-2-ylidene)-9,10-dihydroanthracene-2-carbonyl]- L -alanyl-glycyl- L -alanyl-glycyl- L -alanine ( 1b ): The compound 7 (35 mg, 46 μmol) was added to a solution of KOH 0.2 M in ethanol/H 2 O (9:1, v-v; 5 ml). The mixture reaction was stirred for 120 min at room temperature. After addition of hydrochloric acid until aqueous solution became neutral, the product was extracted with CH 2 Cl 2 (3 × 10 ml). The combined organic layers were dried over Na 2 SO 4 before the solvent was removed in vacuum to yield final product 1b as an orange powder (33 mg, 95%); [ α ] D =99.2 (0.013 M in methanol); 1 H NMR (500 MHz, CD 3 OD): δ 8.25 (s, 1H), 7.86–7.81 (m, 1H), 7.78–7.73 (m, 1H), 7.73–7.66 (m, 2H), 7.33–7.27 (m, 2H), 6.50 (s, 1H), 6.47 (s, 1H), 4.55–4.47 (m, 1H), 4.44–4.31 (m, 2H), 4.05–3.81 (m, 4H), 1.54 (d, 3 J =7 Hz, 3H), 1.52–1.45 (m, 3H), 1.38 (d, 3 J =7 Hz, 3H); 13 C NMR (125 MHz, CD 3 OD): δ 175.0, 174.5, 170.9, 170.2, 139.1, 136.1, 135.6, 135.5, 130.8, 126.1, 125.1, 125.0, 124.6, 120.9, 117.7, 117.3, 51.2, 50.0, 48.8, 42.9, 42.5, 16.8, 16.7, 16.4; HRMS (MALDI; m / z ): [M] + calcd. for C 34 H 33 N 5 O 7 S 4 , 751.1257; found, 751.1252. General method for the preparation of hydrogels In a typical experiment, to 1 ml of 5 × 10 −3 M aqueous solution of 1a or 1b in the presence of 7.5 eq of NaHCO 3 , around 2 mg of the corresponding SWCNTs was added. The suspension was sonicated in an ultrasound bath until a dark red solution was obtained. This process usually took from 30 to 60 min. Low-power ultrasound bath ensures their non-covalent functionalization process, avoiding any significant oxidation stemming from the use of strong and invasive ultrasound equipment. The solution containing the coated 1a /SWCNT or 1b /SWCNT was then centrifuged at low r.p.m. rate (1,500 r.p.m. for 3 min) in an Eppendorf microcentrifuge tube to remove the excess of unfunctionalized SWCNTs that precipitated out. The 75% of the supernatant was recovered from the centrifugation tubes, avoiding sediment at the bottom, and was transferred to a clean tube. Over the dark red solution of 1a /SWCNT or 1b /SWCNT, a few drops of a saturated aqueous solution of CaCl 2 was added, until a hydrogel was formed, obtaining the n / p -nanocomposite 1a /SWCNT/CaCl 2 and 1b /SWCNT/CaCl 2 . For SEM and TEM characterization, the hydrogel was centrifuged for 30 min at 12,000 r.p.m. The supernatant was removed and the concentrated material was washed with deionized water a couple of times, followed by the appropriate treatment describe below. Transmission electron microscopy In the cases where charge screening with CaCl 2 was used to externally control the self assembly, two different methodologies were performed: method A: to a soft basic aqueous solution of 1a /SWCNTs or 1b /SWCNTs, at concentrations in which gels are not formed (<5 × 10 −3 M), CaCl 2 was added. Subsequently, the mixture was drop-casted on Lacey carbon film on 200 mesh copper TEM grids (LC200-Cu). TEM images were obtained after drying the sample by air for 24 h. Method B: in those cases in which charge screening process of nanohybrids’ solutions with CaCl 2 promoted gelling process (concentrations higher than 5 × 10 −3 M) procedures were different. In these cases, concentrated gels were fixed by immersing in an aqueous solution of glutaraldehyde and paraformaldehyde (2.5% and 4%, respectively) for 2 h and then, in an aqueous solution of OsO4 (1%) and potassium ferrocyanide (1.5%) for another 1 h. After washing several times with deionized water, samples were dehydrated by exchange with acetone of increasing concentration (30, 50, 70 up to 100% of acetone). Samples were immersed in each solution for at least 10 min. Gels were included into the epoxy resin precursor and maintained at 80 °C for 2 days for resin’s polymerization. Afterwards, composites were cut in thin films by a microtome for TEM measurements. Scanning electron microscopy SEM images of gels were acquired by using JEOL JSM 6335F microscope working at 10 kV. Before SEM characterization, concentrated gels were fixed by an aqueous solution of glutaraldehyde and paraformaldehyde (2.5% and 4%, respectively) for 2 h. After washing several times with deionized water, sample dehydration was carried out by slow exchanging with a gradient of water–ethanol mixtures (30, 50, 70 up to 100% of ethanol) until the gel was in 100% ethanol. Samples were immersed in each solution for at least 10 min. The ethanol was removed by critical point drying to preserve the structure of the gels for SEM analysis. Dried gels were deposited on graphite and metalized with Au before observation. Atomic force microscopy AFM images were acquired under ambient conditions using SPM Nanoscope IIIa multimode working on tapping mode with a RTESPA tip (Veeco) at a working frequency of ~235 Khz. Height and phase images were simultaneously obtained. The samples were prepared by drop-casting on freshly cleaved mica or highly ordered pyrolytic graphite and were dried under ambient conditions for 24 h. How to cite this article: López-Andarias, J. et al . Controlling the crystalline three-dimensional order in bulk materials by single-wall carbon nanotubes Nat. Commun. 5:3763 doi: 10.1038/ncomms4763 (2014).